Human-induced nitrogen–phosphorus imbalances alter natural and managed ecosystems across the globe The availability of carbon from rising atmospheric carbon dioxide levels and of nitrogen from various human-induced inputs to ecosystems is continuously increasing; however, these increases are not paralleled by a similar increase in phosphorus inputs. The inexorable change in the stoichiometry of carbon and nitrogen relative to phosphorus has no equivalent in Earth’s history. Here we report the profound and yet uncertain consequences of the human imprint on the phosphorus cycle and nitrogen:phosphorus stoichiometry for the structure, functioning and diversity of terrestrial and aquatic organisms and ecosystems. A mass balance approach is used to show that limited phosphorus and nitrogen availability are likely to jointly reduce future carbon storage by natural ecosystems during this century. Further, if phosphorus fertilizers cannot be made increasingly accessible, the crop yields projections of the Millennium Ecosystem Assessment imply an increase of the nutrient deficit in developing regions. The growth of the global demand for phosphorus (P) in a world flooded with reactive nitrogen (N) and CO 2 emitted by human activities is faster than the growth of supply [1] , [2] , [3] , [4] . This creates a N:P imbalance that may induce significant alterations in Earth’s organisms and ecosystems and a P limitation of natural ecosystems growth and agricultural production in the future. The worldwide application of mineral phosphorus fertilizers to croplands is ~17 Tg P per year. When the use of livestock slurry and manure is included, the total phosphorus application in agriculture amounts to 22–26 Tg P per year (ref. 4 ). Unlike nitrogen fertilizers, phosphorus fertilizers are not volatile, so that very little phosphorus is redistributed from croplands to nearby natural terrestrial ecosystems [3] , [4] . However, excessive application of phosphorus fertilizer can result in substantial transfers of phosphorus to adjacent freshwater bodies, followed by transport to coastal waters. In contrast to phosphorus, atmospheric nitrogen deposition from anthropogenic activities is geographically widespread; it mostly impacts northern ecosystems but will likely extend to the tropics during this century [1] . The burning of fossil fuels, and the formation of nitrogen oxides, has resulted in a widespread increase in the deposition of nitrogen, especially around densely populated areas. Globally, the deposition of reactive nitrogen from fossil fuel burning amounts to 25–33 Tg N per year (ref. 4 ). Fertilizer inputs make up a considerable additional amount of ~118 Tg N per year (ref. 4 ). Moreover, the annual human-caused biological fixation of atmospheric N 2 by cultivated leguminous crops and rice is currently estimated at ~65 Tg N per year (ref. 4 ). Only ~22% of these total human inputs of nitrogen ends up accumulating in soils and biomass, whereas ~35% enters the oceans via atmospheric deposition (17%) and leaching via river runoff (18%) [2] . In contrast to these multiple and massive human-caused additions of reactive nitrogen, the only source of atmospheric phosphorus deposition is through mineral aerosols (dust and fly ash from wildfires). This source is small, with a total global flux estimated at ~3–4 Tg P per year (ref. 3 ) and it is not clear whether it will increase or decrease in the future in response to human activities and climate change. In agricultural lands, the use of nitrogen fertilizers has grown more than 10 times since the 1950s, and continues to increase [4] . In contrast, although the use of phosphorus fertilizers tracked that of nitrogen until the 1980s, it has stalled since 1989 (ref. 4 ). The global average N:P ratio of fertilizer inputs has thus increased by 51% since 1975. These global agricultural inputs, however, mask a growing gap in access to phosphorus fertilizers between developed and developing (mainly tropical) countries. Only 10% of the world’s croplands are found in developed countries but they account for 32% of the global nitrogen surplus and for 40% of the phosphorus surplus [5] . As a result of these unbalanced human-induced N and P inputs into the biosphere, the N:P ratio of overall inputs and the N:P ratio of atmospheric deposits, although being extremely variable geographically, have continuously increased in the Northern Hemisphere since pre-industrial times [4] . Future projections of nitrogen emissions suggest an expansion of the area with high anthropogenic nitrogen deposition and high deposited N:P ratios from the populated temperate regions of the Northern Hemisphere into tropical regions [6] . The stoichiometry of these deposits currently presents a molar N:P deposition ratio in the range 44–47 over land, more than twice the current molar ratio in terrestrial plants (22–30) and of 114–370 over the oceans, which is 10–20 times the current molar ratio in marine plankton (~16, the Redfield ratio) [4] . These unbalanced nutrient inputs are very likely to alter the environment and the life it supports. In response to these likely alterations, as phosphorus and its relation with N is pivotal for the functioning of the carbon cycle and thereby also of climate, the question now arises as to whether or not the changes in P and N availability and in N:P ratio can alter the Earth’s capacity to fix carbon from human-induced CO 2 emissions. Coupled climate–carbon cycle models are generally unconstrained by nutrient limitation for land ecosystems and, apart from some models that address potential nitrogen limitations, do not include explicit phosphorus or other soil-nutrient feedbacks on productivity and changes in carbon storage. This lack of soil-nutrient constraint suggests that simulated changes in net primary production (NPP) and increases in vegetation and soil carbon storage in response to rising CO 2 and longer Northern Hemisphere growing seasons are likely over-estimated [7] . Recent progress in implementing mechanistic nitrogen and phosphorus schemes in terrestrial carbon cycle models underscores the importance of nutrient feedbacks, showing reductions in the twenty-first century productivity up to 50% (ref. 8 ). Despite these advances, however, there is large disagreement on the spatial pattern and the strength of future nutrient limitation [9] , and their interaction with the coupled climate–carbon cycle system remains highly uncertain. Here we aim to discern how phosphorus limitations and increased N:P resources will affect the environmental N:P imbalances and the structure, function and diversity of the Earth’s organisms and ecosystems, and in particular future terrestrial ecosystem and cropland productivity and changes in carbon storage, and thereby the function of the carbon cycle. We conduct a literature review of the available observations and experimental evidences of the ecological consequences of human-induced N:P imbalances in the ‘Web of Science’ and conduct a mass balance analysis, that is, we assume a C:N:P ratio and calculate N and P demands for given changes in C pools, for an ensemble of models from the Coupled Climate Carbon Cycle Model Intercomparison Projects (C4MIP and CMIP5) used in the IPCC Fourth and Fifth Assessment Reports. As a result, we report profound and yet uncertain consequences of the human imprint on the phosphorus cycle and N:P stoichiometry for the structure, functioning and diversity of terrestrial and aquatic organisms and ecosystems. We show that limited phosphorus and nitrogen availability are likely to jointly reduce future carbon storage by natural ecosystems during this century, and that if phosphorus fertilizers cannot be made increasingly accessible, the crop yields projections of the Millennium Ecosystem Assessment imply an increase of the nutrient deficit in developing regions. Environmental N:P imbalances Our review of the literature showed that the higher increases of N inputs than of P inputs into the biosphere ( Figs 1 and 2 ) result in increases in N:P deposition rates especially in the Northern hemisphere ( Fig. 3 ), and that, as a result, most studies reported increases in the N:P ratio of soils and waters ( Fig. 4 ). Increases in nitrogen deposition have increased the N:P ratios of soils in terrestrial ecosystems in the temperate zone, in northern and central Europe and in North America ( Fig. 4 ). Increases in nitrogen deposition have also been observed in some tropical regions [10] , areas that, despite being complex and heterogeneous, are usually less nitrogen-limited than temperate regions. Some recent studies have already observed increases in soil N:P ratios due to N deposition in tropical forest [11] . 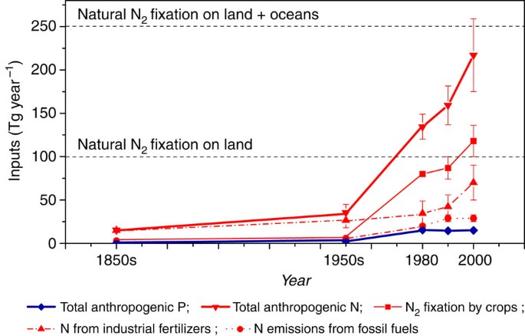Figure 1: Anthropogenic N and P inputs to the biosphere. Anthropogenic reactive nitrogen and phosphorus inputs to the biosphere (mean±s.e., Tg per year) since the industrial revolution (1860). Error bars indicate the range of the data reported4. Figure 1: Anthropogenic N and P inputs to the biosphere. Anthropogenic reactive nitrogen and phosphorus inputs to the biosphere (mean±s.e., Tg per year) since the industrial revolution (1860). Error bars indicate the range of the data reported [4] . 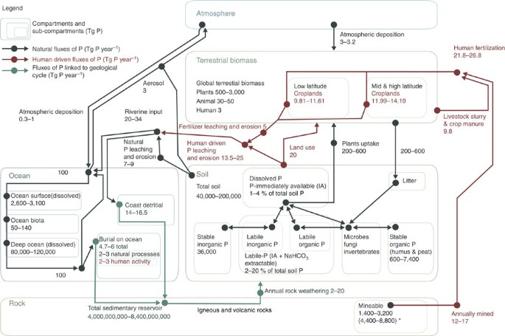Figure 2: Updated phosphorus cycle. Updated data on the amount of phosphorus (Tg P) in the different Earth compartments and on the annual natural and human-driven annual fluxes (Tg P per year) among these different compartments. References used to update the data are also depicted (References inSupplementary Table S21). Potential reserves (now not profitable under current prices, but exploitable in the future with better technology and higher market prices for phosphorus). ‘Land use’ includes an estimation of all human activities (changes in land use, crop management and deforestation) that increase phosphorus mobilization from humus to stream water (initial mobilization less the part that is accumulated again on land) where thereafter this phosphorus mobilized can be loaded in continental waters or taken up by plants70. Full size image Figure 2: Updated phosphorus cycle. Updated data on the amount of phosphorus (Tg P) in the different Earth compartments and on the annual natural and human-driven annual fluxes (Tg P per year) among these different compartments. References used to update the data are also depicted (References in Supplementary Table S21 ). Potential reserves (now not profitable under current prices, but exploitable in the future with better technology and higher market prices for phosphorus). ‘Land use’ includes an estimation of all human activities (changes in land use, crop management and deforestation) that increase phosphorus mobilization from humus to stream water (initial mobilization less the part that is accumulated again on land) where thereafter this phosphorus mobilized can be loaded in continental waters or taken up by plants [70] . 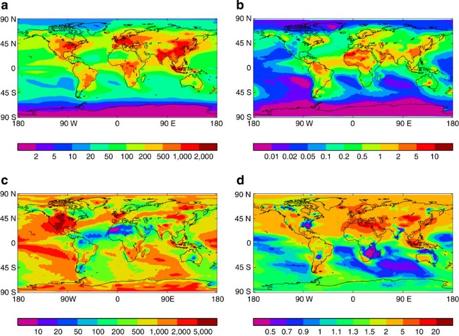Figure 3: Increasing N:P ratio of atmospheric depositions. (a) Total nitrogen and (b) total phosphorus deposition (mg m−2per year), 2000–2010, (c) ratio of deposited N to deposited P, for the 2000–2010 decade and (d) ratio of the deposited N:P ratio between 2000–2010 decade and 1850. Data are from Lamarqueet al.6and Mahowaldet al.3Only phosphorus as phosphate is considered. Full size image Figure 3: Increasing N:P ratio of atmospheric depositions. ( a ) Total nitrogen and ( b ) total phosphorus deposition (mg m −2 per year), 2000–2010, ( c ) ratio of deposited N to deposited P, for the 2000–2010 decade and ( d ) ratio of the deposited N:P ratio between 2000–2010 decade and 1850. Data are from Lamarque et al. [6] and Mahowald et al. [3] Only phosphorus as phosphate is considered. 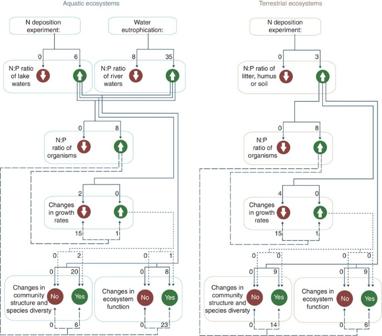Figure 4: Ecological effects of increased environmental N:P ratios. Number of ‘Web of Science’ studies reporting effects of increased environmental nitrogen availability on increased environmental N:P ratios, number of studies reporting effects of increased environmental N:P ratios on increased organism’s N:P ratios, decreased growth rates and changes in community structure and ecosystem functioning, number of studies reporting effects of increased organism’s N:P ratios on decreased growth rates and changes in community structure and ecosystem functioning, and number of studies reporting effects of decreased growth rates on changes in community structure and ecosystem functioning (References inSupplementary Tables S1–S18). Effects of nitrogen deposition and eutrophication and increased environmental N:P ratios are indicated by continuous lines, effects of increased organisms’ N:P ratios by dashed lines and effects of increased growth rates by dotted lines. Full size image Figure 4: Ecological effects of increased environmental N:P ratios. Number of ‘Web of Science’ studies reporting effects of increased environmental nitrogen availability on increased environmental N:P ratios, number of studies reporting effects of increased environmental N:P ratios on increased organism’s N:P ratios, decreased growth rates and changes in community structure and ecosystem functioning, number of studies reporting effects of increased organism’s N:P ratios on decreased growth rates and changes in community structure and ecosystem functioning, and number of studies reporting effects of decreased growth rates on changes in community structure and ecosystem functioning (References in Supplementary Tables S1–S18 ). Effects of nitrogen deposition and eutrophication and increased environmental N:P ratios are indicated by continuous lines, effects of increased organisms’ N:P ratios by dashed lines and effects of increased growth rates by dotted lines. Full size image In several lakes of Europe and eastern North America, the two regions which have been exposed to the highest nitrogen deposition over the past century, increases in N:P ratios have paralleled shifts from a nitrogen-limited to a phosphorus-limited environment [12] . In coastal waters, the amounts of anthropogenic nutrients received from agricultural areas through rivers have increased in recent decades [13] , leading to observations of higher N:P ratios in the waters off the coasts of China and South America, and in the North Atlantic and the Baltic Sea [14] , [15] . However, decreases in the coastal water N:P ratios have also been reported, especially for estuaries in emerging economies characterized by growing agricultural inputs of phosphorus, such as Turkey [13] and Mexico [13] . In the open ocean, the increases in the N:P ratios of the atmospheric inputs ( Fig. 3 ) enlarge the extent of phosphorus-limited areas [13] . Phosphorus fertilizer continues to be overused in croplands of developed countries, causing eutrophication of downstream ecosystems, but it is not applied in sufficient amounts in developing countries, where food security is a challenge [16] . In contrast to the global tendency for an enhancement of the N:P ratio, intensely used pastoral areas and areas where animal slurry is used as fertilizer [17] are being polluted with excess phosphorus; this phosphorus decreases the N:P ratio of water in soil, lakes and streams. In contrast, where crops are fertilized solely with industrial fertilizers, streams and lakes have systematically shown high N:P ratios [18] . Impacts of N:P ratio imbalances on organisms and ecosystems An increasing number of studies report increases in the N:P ratio of terrestrial and aquatic plants in response to increased nitrogen loadings ( Fig. 4 ) ( Supplementary Tables S1–S18 ). The literature review shows that nitrogen deposition (or any type of nitrogen loading) has direct effects on organisms and ecosystem structure and function by itself, but also affects them indirectly through alteration of the N:P ratio [19] ( Fig. 4 ) ( Supplementary Tables S1–S18 ); various metabolic processes are thereby affected to different degrees. For example, the maximum growth rate capacity of organisms is characterized by a specific ratio of RNA to protein; and this ratio has been related to the organisms’ N:P ratio [20] . In the Mediterranean shrub Erica multiflora , for instance, increases in N:P ratio were accompanied by decreased proportions of primary metabolites (sugars, amino acids) relative to lipids and secondary metabolites, and also by lower growth rates [21] . Several studies have observed that the N:P ratio of foliage correlates negatively with net photosynthetic rate [22] , plant growth [23] and biomass production [24] ( Fig. 4 ) ( Supplementary Tables S1–S18 ). The increases in N:P ratio of environment and organisms thus produce a cascade of effects favouring organisms with lower growth rates and changing communities species compositions and function ( Fig. 4 ) (see details in Supplementary Tables S1–S18 ). The N:P ratio has thus also been found to be significantly related to plant community composition and diversity [19] , [25] , but with different sign depending on the study. N:P ratios are often correlated negatively with diversity [26] but there is also evidence suggesting precisely the opposite—that N:P stoichiometry is related positively to species diversity. For example, Laliberte et al. [27] showed recently that increasing phosphorus limitation along long-term soil chronosequences occurs in parallel with a continual increase in vascular plant diversity. Declines in diversity owing to nitrogen deposition can also be due to other factors linked to nitrogen deposition, than the change in N:P ratio itself [28] . In fact, nitrogen deposition could promote plant diversity, because rare species are favoured under phosphorus-limited conditions [29] . The relationship between N:P stoichiometry and species diversity [30] is, moreover, not necessarily linear. For instance, Sasaki et al. [25] have shown unimodal relationships between N:P stoichiometry and species richness in terrestrial ecosystems that reach a maximum at ~20 biomass N:P ratio, that is, at a much lower ratio than current deposition ratios [4] . Several important ecosystem processes such as the energy and element transfers through trophic levels have also been related to these changes in organism’s N:P ratios [30] ( Fig. 4 ) (see details in Supplementary Tables S1–S18 ). Among these ecosystem processes, the fixation of CO 2 is also likely to be affected by the changes in P and N availabilities and the corresponding changes in the N:P ratio, even though reduced growth does not necessarily mean reduced C storage (for example, there is a decline in litter decomposition rates following atmospheric nitrogen deposition [31] in northern ecosystems, leading to an accumulation of carbon in the forest floor). Capacity of terrestrial ecosystems to fix CO 2 Using the Coupled Climate Cycle Model Intercomparison Projects (C4MIP and CMIP5), we observed that in the absence of nutrient limitation, terrestrial NPP increased between 2000 and 2099 by 3–57 Pg C per year for the C4MIP model ensemble ( n =22) ( Supplementary Fig. S1 ) and −4 to 12 and 10–64 Pg C per year for CMIP5 representative concentration pathways (RCP) 2.6 and 8.5, respectively (for the CMIP5 ensemble, see Supplementary Table S20 ). The change in NPP generally resulted in increased carbon storage in both vegetation biomass (+22 to +477 Pg C for C4MIP and −369 to +435 Pg C for CMIP5) and soils (−45 to +457 Pg C and −85 to 324 Pg C for C4MIP and CMIP5, respectively, Supplementary Figs S1 and S2 ) by 2099. The majority of models show high sensitivity of productivity to CO 2 because they all lack P limitation and all but two models lack N limitation. Because of the slow rate of phosphorus release from weathering, compared with losses from erosion, leaching and occlusion, our analysis of the capacity of terrestrial ecosystems to fix carbon from human-induced CO 2 emissions ( Supplementary Tables S19-S21 and Supplementary Figs S1 and S2 ) suggested that phosphorus limitation will be met first and nitrogen limitation second in most regions ( Fig. 5 ). Globally, the increase in nutrient availability needed to sustain the carbon stock changes projected by the C4MIP models, ranged from −0.9 to 6.2 Pg P and −4.9 to 36.7 Pg N for the coupled simulations and from 0.8 to 9.2 Pg P and 4.7 to 53.9 Pg N for the uncoupled simulations (positive numbers indicate a higher demand; Fig. 5a ). For the CMIP5 models, the change in nutrient availability needed to sustain the carbon stock changes, ranged from −0.9 to 4.3 Pg P and −5.4 to 25.1 Pg N for the RCP 2.6 (the lower projection for fossil fuel emissions) and from −1.7 to 6.5 Pg P and −10.0 to 38.6 Pg N for the higher fossil fuel (RCP 8.5) scenario ( Fig. 5b ). In comparison, the size of the global plant-accessible labile-phosphorus soil pool is only 13.2 Pg P (estimated as the mean of the range in the labile phosphorus pool in Fig. 2 ). The lower demand, and for few models a negative demand, for the coupled models was due to lower soil or vegetation carbon stocks from increased soil organic matter decomposition or from increased mortality due to climate stress. 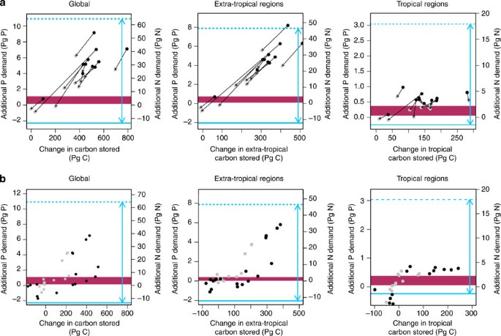Figure 5: P and N demand for changes in land carbon stocks. Estimated phosphorus and nitrogen demand for changes in land carbon stocks from 2000 to 2099 for global and regional analyses from the results of (a) the C4MIP uncoupled models (where climate feedbacks from fluxes of land and ocean carbon to the atmosphere were excluded) and the coupled models (where climate feedbacks from fluxes of land and ocean carbon to the atmosphere were included), and (b) the CMIP5 models. The horizontal lines indicate the estimated supply of phosphorus (blue, solid and dashed) and nitrogen (maroon) in the year 2100 considering cumulative changes in nitrogen and phosphorus inputs. For nitrogen, the range of uncertainty (thickness of the line) represents uncertainty from N-inputs and losses (ignoring the dynamics of the total labile pool), whereas with P the uncertainty (distance between solid and dashed lines) represents two different assumptions on the labile P pool and it being available (dashed blue line) or unavailable, due for example to competition with microbes (solid blue line) for uptake by plants (Supplementary MethodsandSupplementary Table S19). The negative values for the lower P threshold indicate a decrease in immediately available P due to gross losses from leaching and occlusion being slightly larger than gross inputs from weathering (ignoring changes in the labile pool of P). Circles above the blue lines indicate that models predict that the phosphorus demand will not be met. The C4MIP models are: TAXIS, HadCM3, IPSL-CM2, IPSL-CM4-LOOP, CSM, MPI, LLNL, FRCGC, UMD, UVIC, CLIMBER and BERNCC and the 35 CMIP5 models are listed inSupplementary Table S2. Grey points foraare for the coupled C4MIP models and the black points for the uncoupled C4MIP models, whereas the grey points forbare for RCP 2.6 and the black points for RCP 8.5. Figure 5: P and N demand for changes in land carbon stocks. Estimated phosphorus and nitrogen demand for changes in land carbon stocks from 2000 to 2099 for global and regional analyses from the results of ( a ) the C4MIP uncoupled models (where climate feedbacks from fluxes of land and ocean carbon to the atmosphere were excluded) and the coupled models (where climate feedbacks from fluxes of land and ocean carbon to the atmosphere were included), and ( b ) the CMIP5 models. The horizontal lines indicate the estimated supply of phosphorus (blue, solid and dashed) and nitrogen (maroon) in the year 2100 considering cumulative changes in nitrogen and phosphorus inputs. For nitrogen, the range of uncertainty (thickness of the line) represents uncertainty from N-inputs and losses (ignoring the dynamics of the total labile pool), whereas with P the uncertainty (distance between solid and dashed lines) represents two different assumptions on the labile P pool and it being available (dashed blue line) or unavailable, due for example to competition with microbes (solid blue line) for uptake by plants ( Supplementary Methods and Supplementary Table S19 ). The negative values for the lower P threshold indicate a decrease in immediately available P due to gross losses from leaching and occlusion being slightly larger than gross inputs from weathering (ignoring changes in the labile pool of P). Circles above the blue lines indicate that models predict that the phosphorus demand will not be met. The C4MIP models are: TAXIS, HadCM3, IPSL-CM2, IPSL-CM4-LOOP, CSM, MPI, LLNL, FRCGC, UMD, UVIC, CLIMBER and BERNCC and the 35 CMIP5 models are listed in Supplementary Table S2 . Grey points for a are for the coupled C4MIP models and the black points for the uncoupled C4MIP models, whereas the grey points for b are for RCP 2.6 and the black points for RCP 8.5. Full size image The extra amount of phosphorus needed to sustain the increased carbon storage exceeded all plausible phosphorus supply scenarios by the end of the twenty-first century for all of the 22 coupled and uncoupled simulations, and all of the 35 CMIP5 models ( Fig. 5a,b ). This estimation assumed no additional plant uptake of plant-available labile phosphorus, which is consistent with observations that microbes currently sequester much of this labile phosphorus [32] . Assuming that the labile-phosphorus soil pool could become entirely accessible for plant uptake, sufficient phosphorus would be available in most of the coupled model runs ( Fig. 5a,b ) under this ‘most optimistic’ supply scenario. At this global scale, the extra amount of nitrogen needed to sustain the increased carbon storage exceed all plausible nitrogen supply scenarios by the end of twenty-first century for 18 out of 22 coupled and uncoupled simulation and 11 out of the 35 CMIP5 models. At the regional scale, the change in tropical ecosystem phosphorus demand ( Fig. 5 ) was largely driven by changes in vegetation carbon. Because of the high C:P ratio of woody biomass, this carbon sink imposes only a relatively small phosphorus demand (compared with the demand associated with changes in soil carbon stocks). The size of the tropical labile-phosphorus pool (3.3 Pg P; Supplementary Tables S19–S21 and Supplementary Figs S1 and S2 ) may suffice to compensate for the smaller cumulative inputs of phosphorus from weathering (0.11 Pg P) and dust deposition (0.03 Pg P) relative to phosphorus losses through erosion, leaching and occlusion (0.39 Pg P; Supplementary Tables S19–S21 and Supplementary Figs S1 and S2 ) over the same time period. We estimated an extra-tropical labile pool of 9.9 Pg P (from a global labile-phosphorus pool of 13.2 Pg P), three times as high as the tropical labile-phosphorus pool, with cumulative (over the years 2000–2099) extra-tropical dust and weathering inputs at 1.4 Pg P but exceeded by large leaching and occlusion losses at 3.4 Pg P. Crop yields For the analysis in croplands, the change in crop production (including wheat, rice, maize, roots/tubers and pulse and non-biofuel oil crops) projected by the Millenium Ecosystem Assessment went from 1,568 Tg C per year in 2000 to 2,475 Tg C per year in 2050. This suggests an increase in phosphorus demand from 12.3 Tg P per year to 18.9–19.9 Tg P per year, across the four Millenium Ecosystem Assessment scenarios, and in nitrogen demand from 81 Tg N per year to 135.6–142.5 Tg N per year (taking C:P and C:N stoichiometry of crops as a model; Supplementary Table S19 ). Integrating over the cumulative additions of phosphorus from 2000 to 2050, and 2000 to 2100, we estimated that applications of 1,232 Tg P and 3,195 Tg P would be needed, respectively, to satisfy this increasing demand. Our analyses show that the future phosphorus deficits for cereal crops (including wheat, maize and rice) may be especially large in Africa and Russia where the potential yields are not realized ( Fig. 6 ). 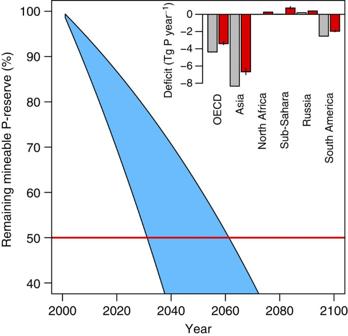Figure 6: Projected depletion of mineable P. Expected depletion of mineable phosphorus to satisfy total crop phosphorus demand throughout the twenty-first century. Inset indicates the deficit of phosphorus under current (year 2000, grey bars) and projected future (year 2050, red bars) balances between cereal crop phosphorus-demand and supply (positive values) or a surplus of phosphorus in negative values. For the year 2040, at current rates of phosphorus application, phosphorus surpluses decrease and phosphorus deficits increase indicating the likely increase in the application of finite phosphorus reserves (with error bars representing the max–min range from the Millennium Ecosystem Assessment cereal yield storylines). It is likely that the mineable phosphorus pool (blue shaded area; not considering additional potential reserves, seeFig. 1) will be depleted by over 50% (horizontal red line) by mid-late twenty-first century. Figure 6: Projected depletion of mineable P. Expected depletion of mineable phosphorus to satisfy total crop phosphorus demand throughout the twenty-first century. Inset indicates the deficit of phosphorus under current (year 2000, grey bars) and projected future (year 2050, red bars) balances between cereal crop phosphorus-demand and supply (positive values) or a surplus of phosphorus in negative values. For the year 2040, at current rates of phosphorus application, phosphorus surpluses decrease and phosphorus deficits increase indicating the likely increase in the application of finite phosphorus reserves (with error bars representing the max–min range from the Millennium Ecosystem Assessment cereal yield storylines). It is likely that the mineable phosphorus pool (blue shaded area; not considering additional potential reserves, see Fig. 1 ) will be depleted by over 50% (horizontal red line) by mid-late twenty-first century. Full size image The available data thus shows that the unbalanced human-induced inputs of carbon, nitrogen and phosphorus into the biosphere are altering environmental N:P ratios and that these altered environmental N:P ratios are affecting the metabolism and growth rates, and therefore the life histories and competitiveness of various microbes, plants and animals [33] . The observed metabolic shifts associated with organisms N:P ratio change [21] provide support for the hypothesis that exceedances of the optimal N:P ratios can reduce growth rates [34] . Several studies have verified this hypothesis in diverse unicellular organisms, zooplankton and fish in aquatic ecosystems; there is evidence that this hypothesis can also be extended to a large number of terrestrial plants and animals, albeit with a few exceptions [35] ( Fig. 4 ). The observed increasingly imbalanced inputs of N and P require substantial upregulation of the homoeostatic and flexibility mechanisms of the different organisms and communities and their corresponding energy costs, and in some cases it is likely that they will exceed the homoeostatic and flexibility limits, that is, the limits in the imbalance of the inputs of N and P that these homoeostatic and flexibility mechanisms can cope with [36] . Organisms and communities present a certain degree of homoeostasis, a certain capacity to maintain roughly constant stoichiometries by adapting their functioning and by acquiring more of the limiting nutrients. However, the homoeostatic capacity and the ranges of stoichiometric flexibility of organisms and communities are limited, and differ among species. The species that are stoichiometrically more homoeostatic than others tend to have higher biomass; and ecosystems dominated by more homoeostatic species tend to have higher productivity and stability [37] . Less homoeostatic species tend to have greater nitrogen and phosphorus concentrations and lower N:P ratio [38] . This suggests that fast shift rates of N:P ratio can be more detrimental for less homoeostatic species, with consequences for community composition and carbon cycling. The changes in community composition in response to altered N–P availability by nitrogen enrichment can result from multiple processes. These are some reported examples: First, the N 2 -fixing community loses its competitive advantage over other species and decreases in abundance [39] . Second, increased N:P availability ratio in soils and waters favours the slow-growing species with high optimal N:P ratios at the expense of the fast-growing species with lower optimal N:P ratio [34] . Third, by favouring species with slower growth rates, food sources with higher N:P ratios decrease the rates of energy transfer through food webs [40] , favouring shorter trophic webs with fewer predators [41] , thus potentially decreasing biodiversity. Fourth, in phosphorus-limited zones of the coastal waters, zooplankton (for example, copepods) adapt their feeding behaviour to counteract the resource limitation in selecting higher phosphorus-containing organisms (for example, ciliates) rather than nutrient-limited phytoplankton [42] . Fifth, in the open ocean, altered nutrient input ratios reduce food-web diversity, alter phytoplankton community composition and could increase toxic blooms of phytoplankton [43] . Looking at the past may reveal how changes in the N:P ratio influence marine biota. Diatom frustule size seems to have decreased through the Neogene, linked with a decrease in phosphorus availability [44] . Further back in time, large episodic accumulations of phosphorite in the early Paleozoic, Permian, Jurassic, early Cretaceous and Cenozoic periods [45] indicate periods of well-suited sedimentation conditions combined with a high biological productivity, potentially driven by enhanced delivery of P by continental weathering. Most of these events were associated with widespread anoxic conditions, sea-level changes, tectonics and biodiversification [44] , [45] , [46] , [47] . For example, phytoplankton adapted to phosphorus-rich environments is thought to have diversified during the early Palaeozoic in open waters overlying deeper anoxic zones [48] . Enhanced phosphorus content compared with nitrogen, however, does not necessarily confer benefits to the marine biomass. An example is the possible decline in growth efficiency and animal biomass in benthic marine ecosystems in the Triassic, which led to a slow recovery after the Permian mass extinction that coincided with a period of supposed low-nitrogen but high-phosphorus delivery to the ocean [49] . Marine ecosystems in the geological past thus appear to have been highly sensitive to changes in the N:P ratio, although most events recorded a decrease in this ratio during transition periods ranging from 10 4 to 10 6 years. A strong increase in this ratio over a few decades, as is now occurring in response to human activities, seems unprecedented in Earth’s history. The imbalanced human-induced inputs of N and P are also affecting the functioning of ecosystems. For many regions of the Northern Hemisphere, human nitrogen inputs are converting originally nitrogen-limited ecosystems into a state of nitrogen saturation, with nitrogen losses to aquatic ecosystems and with high rates of nitrogen volatilization [50] . The response of tropical ecosystems to nitrogen addition is more uncertain. Some models suggest that tropical forests will be unresponsive to nitrogen enrichment because it is already plentiful and phosphorus is the key limiting nutrient [8] , [51] . However, the diversity of conditions with nutrient limitation is very high in tropical forests [52] , [53] , and therefore uncertainty is large. Furthermore, increased nitrogen loadings can affect ecosystem phosphorus cycling, as observed in a wide variety of terrestrial ecosystems [54] , by favouring higher plant phosphorus uptake e.g. through enhanced activity of soil phosphatases [55] , root phosphatases [56] or changing symbiotic fungi [57] . Nonetheless, in the long term, these mechanisms seem quantitatively insufficient to deliver enough phosphorus to alleviate phosphorus limitation [58] . On the other hand, eventual negative effects of deposited NH 4 + on litter decomposition, as frequently observed in northern ecosystems [31] , could slow nutrient cycling and further reduce phosphorus availability and ecosystem productivity. Few studies have focused on the role of changes in atmospheric deposition or riverine input of nutrients (including phosphorus) on marine biota and productivity. Krishnamurthy et al. [59] have shown that changes in the deposition of atmospheric nitrogen and phosphorus should only have a weak effect on marine productivity and the marine carbon sink on a global scale, because these depositions are small relative to the input of these nutrients from deeper waters by ocean mixing and upwellings. However, the potential for compensatory effects of these changes in nutrient input with the expected decrease in the vertical supply of phosphorus from deep water due to marine stratification [60] remains largely unknown. Because anthropogenic riverine supply and atmospheric deposition are concentrated near coasts, it is the coastal zone that is most affected by phosphorus changes on short timescales [61] . The responses of communities and ecosystems to environmental change are likely to be more complicated than predicted from N and P alone or the ratios between them. There are many complexities in ecosystem functioning including multiple factors and nutrients limiting productivity: for example, nitrogen deposition also depletes ecosystems of calcium as soils are acidified, promoting calcium limitation (for example, in northern temperate forests), while there is evidence that N, P and K all limit different components of biomass production in lowland tropical rain forests [53] . However, analysing C:N:P interactions and the isolation of the N:P impacts in our analysis is already one important step ahead with respect to previous studies. The mass balance approach used here shows that limited P and N availability are likely to jointly reduce future carbon storage by terrestrial ecosystems during this century. A high sensitivity to model assumptions was found in this study, indicating that the future mobilization of phosphorus stocks, in particular soil phosphorus and interactions with microbial processes is critical for sustaining changes in future carbon stocks. Unfortunately, current process understanding is lagging behind model needs [8] , [58] . Knowledge about the potential for ecosystems to tap into the labile-phosphorus pool and for nitrogen deposition to affect the processes by which plants may try to take up phosphorus from the labile pool appears crucial to determine the future carbon sequestration potential of terrestrial ecosystems and specially of tropical ecosystems. For the extra-tropical regions ( Fig. 5 ), the calculated change in phosphorus supply was insufficient to support the projected changes in carbon stocks. This was mainly due to increases in P bound in soil carbon, which tends to have a lower C:P ratio than vegetation. This result is somewhat surprising given the paradigm that non-tropical systems are considered less phosphorus-limited than tropical systems [62] but consistent with more recent work suggesting equal nutrient limitation across biomes [63] and near future shifts from N to P limitations at high latitudes although nutrient limitations in the tropics decline [8] . The magnitude of the marine sink of anthropogenic CO 2 is more certain than the terrestrial sink [64] and can be assessed using several methods, now all converging towards a figure of 2.4±0.5 Pg C per year (ref. 65 ). The marine sink is mostly due to physical and chemical mechanisms. It is mainly driven by increasing levels of atmospheric CO 2 , which tend to increase diffusion in regions that exhibit natural CO 2 uptake (for example, North Atlantic) and to decrease outgassing in regions that experience natural CO 2 outgassing (for example, equatorial Pacific). Thus, contrary to what happens on land, no additional phosphorus input is required to absorb most of the anthropogenic carbon fixed in the oceans. However, any increase or reduction of phosphorus input to the oceans from atmospheric deposition or from rivers potentially affects biological carbon fixation in the oceans and indirectly perturbs air-sea CO 2 fluxes – but these effects are still largely unknown. In the oceans, with low living-biomass relative to its annual turnover, the carbon and nutrient cycles are tightly coupled. With rapid recycling of carbon and nutrients, the ocean carbon–climate feedback seems weak at the century timescale, but a remaining question is whether the changes in the C:N:P ratios in both the particulate and dissolved organic matter pools may provide a mechanism for biological processes to change the amount of carbon sequestered by the ocean [66] . A recent study [67] suggests that coastal oceans are an anthropogenic sink of CO 2 of 0.2 Pg C per year and that it is mainly due to phosphorus and nitrogen increasing accompanied by usually also increasing N:P ratios, biological activity and burial of carbon in organic shelf-sediments, but not in open ocean. At crop level, our results would mean that mineable phosphorus reserves would be depleted by over 100% by 2100 given the lower and upper estimates for these reserves from Fig. 2 . We observed that future phosphorus deficits for cereal crops (including wheat, maize and rice) may be especially large in Africa and Russia where the potential yields are not realized ( Fig. 6 ), which is in agreement with previous work [68] and which has large implications for the sustainability of global agriculture, and its geopolitical consequences. In conclusion, a key and complex impact of the N:P ratio can be anticipated in a carbon- and nitrogen-enriched current and future world. The many lines of evidence reported here indicate that the changes in phosphorus and N:P ratios are, and will become more so, vital through their controlling role on organism and ecosystem functioning and structure, the carbon cycle, climate and agriculture. Nevertheless, we still have little knowledge of where, how and to what degree the imbalance in phosphorus and nitrogen additions to ecosystems will affect the structure and diversity of microbial, plant and animal communities, and their functioning, including for example organic matter decomposition, N 2 fixation, N 2 O and NO x emissions or CO 2 uptake, and the magnitude of the feedback of this altered Earth-system structure and functioning on nutrient cycling and climate change. However, our estimations indicate that the change in nitrogen and phosphorus supply is likely insufficient to support the projected changes in carbon stocks even for the extra-tropical regions, which is surprising because non-tropical systems are considered less phosphorus-limited than tropical systems. Observational and experimental ecological evidences To check the current impacts of the shifts in N:P ratio by human driven eutrophication, we reviewed the ‘Web of Science’ database until December 2012. We summarized the studies reporting: effects of increased environmental nitrogen availability on soil and water N:P ratios, the effects of environmental N:P ratios on organism’s N:P ratios, growth rates and changes in community structure and ecosystem functioning, the effects of organism’s N:P ratios on growth rates and changes in community structure and ecosystem functioning and the effects of growth rates on changes in community structure and ecosystem functioning ( Fig. 4 ). Terrestrial nutrient constraints on carbon sequestration We applied a mass balance approach underpinned by fixed C to nutrient stoichiometries for an ensemble of models from the Coupled Climate Carbon Cycle Model Intercomparison Projects (C4MIP and CMIP5) used in the IPCC Fourth and Fifth Assessment Reports. Two sets of C4MIP model simulations were analysed, the first set included ‘uncoupled’ simulations where climate feedbacks from fluxes of land and ocean carbon to the atmosphere were excluded (these models have a higher marine and terrestrial carbon sink being caused by elevated CO 2 alone), and a second set of ‘coupled’ simulations where climate change is influenced by fossil fuel emissions and land and ocean carbon feedbacks [64] . For the CMIP5 experiment, we analysed changes in nutrient demand for the Representative Concentration Pathways 2.6 and 8.5, which correspond to a year 2100 CO 2 concentration of 421 and 936 μmol mol −1 . The RCP 2.6 scenario reaches a radiative forcing of 2.6 W m −2 in 2100, with a peak in CO 2 concentrations in 2050, followed by a decline [69] . Stoichiometric mass balance approaches are commonly used to evaluate coupled carbon-nutrient cycling at multiple scales spanning from leaf to globe [7] , [8] . Here, the approach of Hungate et al. [7] was adapted to evaluate potential phosphorus and nitrogen limitation globally, as well as separately for tropical, extra-tropical and cropland regions. We first estimated the change in phosphorus and nitrogen demand from the modelled increases in vegetation and soil carbon stocks in natural ecosystems and croplands between 2000 and 2099. Then, this demand was confronted with corresponding scenarios of changes in phosphorus and nitrogen supply ( Supplementary Tables S19 and S20 , Supplementary Figs S1 and S2 and Supplementary Method s ). How to cite this article: Peñuelas, J. et al. Human-induced nitrogen–phosphorus imbalances alter natural and managed ecosystems across the globe. Nat. Commun. 4:2934 doi: 10.1038/ncomms3934 (2013).